A new phyllopod bed-like assemblage from the Burgess Shale of the Canadian Rockies Burgess Shale-type fossil assemblages provide the best evidence of the ‘Cambrian explosion’. Here we report the discovery of an extraordinary new soft-bodied fauna from the Burgess Shale. Despite its proximity ( ca . 40 km) to Walcott’s original locality, the Marble Canyon fossil assemblage is distinct, and offers new insights into the initial diversification of metazoans, their early morphological disparity, and the geographic ranges and longevity of many Cambrian taxa. The arthropod-dominated assemblage is remarkable for its high density and diversity of soft-bodied fossils, as well as for its large proportion of new species (22% of total diversity) and for the preservation of hitherto unreported anatomical features, including in the chordate Metaspriggina and the arthropod Mollisonia . The presence of the stem arthropods Misszhouia and Primicaris , previously known only from the early Cambrian of China, suggests that the palaeogeographic ranges and longevity of Burgess Shale taxa may be underestimated. Burgess Shale-type deposits are critical to our understanding of the ‘Cambrian explosion,’ because their soft-bodied biotas offer far more palaeobiological and palaeo ecological information than is typically available from the fossil record [1] . A century of intensive collecting has revealed that these exceptionally preserved biotas (c. 45) occur globally [2] , yet most are characterized by relatively low-diversity faunas. Despite this effort, Walcott’s original Burgess Shale locality, the phyllopod bed [3] , remains unmatched for its exquisite preservation, exceptional high diversity and abundance of soft-bodied taxa within a narrow stratigraphic interval [4] , [5] . Whether this assemblage is typical of Cambrian marine communities, however, remains an open question [6] . The early Cambrian Chengjiang biota is also distinguished by a high diversity of soft-bodied taxa, many of which are unique to that deposit, and by the preservation of key anatomical features that provide particular insights into the origins of animal bodyplans [7] . Despite concerted collection efforts, our understanding of the global evolutionary and ecological signals of the Cambrian ‘explosion’ is nonetheless hindered by the scarcity and limited temporal distribution of well-preserved, abundant and diverse Burgess Shale-type fossil assemblages. Here we report the discovery of arguably the most significant new Cambrian Burgess Shale-type fossil assemblage since that of the Chengjiang biota in 1984 (ref. 8 ). The soft-bodied fossil assemblage is noteworthy for its high proportion of new taxa—which is surprising considering the locality’s close geographical and temporal proximity to the Walcott Quarry—and also for the preservation of previously unknown or unreported anatomical features, and for the presence of taxa previously only known from the early Cambrian of China. Age and palaeoenvironmental setting The new assemblage, discovered in 2012, occurs ca. 40 km southeast of Walcott’s Quarry in northern Kootenay National Park ( Supplementary Fig. 1 ), in multiple exposures of a 2-m horizon of fine-grained claystones near the top of the Stephen Formation ( Figs 1 , 2 ). This stratigraphic position and the trilobite fauna indicate that this is the youngest assemblage yet identified from the Burgess Shale ( Fig. 2 and Supplementary Note 1 ). Local stratigraphic evidence confirms that the Marble Canyon assemblage, like the Walcott Quarry and most other soft-bodied assemblages of the Burgess Shale [9] , occurs in direct association with the Cathedral Escarpment, a major break in submarine topography ( Supplementary Note 1 ). The new assemblage was preserved on the offshore margin of the escarpment, less than 3,000 m west of the locality at Stanley Glacier [10] , the only soft-bodied fossil assemblage presently known from atop the Cathedral Escarpment, in the ‘thin’ Stephen Formation [11] . As in the Walcott Quarry [4] , proximity to the escarpment promoted rapid entombment of fossil assemblages within or close to their original habitats. A distinct shallow-tier, low-diversity trace fossil assemblage that is unlike that of other Burgess Shale-type deposits is preserved in close vertical proximity to soft-bodied fossils ( Supplementary Figs 3–5 ), suggesting that periodic oxygenated conditions developed during deposition of the fossil-bearing interval [12] , [13] . A low-diversity shelly fossil assemblage occurs in associated carbonate facies ( Supplementary Fig. 6 ) and may reflect transport from shallower water environments. 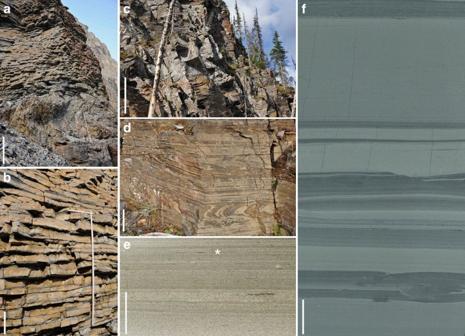Figure 1: Sedimentary facies. Sedimentary facies of the Stephen Formation at the Marble Canyon locality. (a,b) Carbonate mudstone and wackestone facies; (c–f) Shale facies. (a) Outcrop of carbonate mudstone and wackestone facies showing 2.25 m slump fold in lower field of view, ~30 m above base of the Stephen Formation. (b) Outcrop of carbonate mudstone and wackestone facies showing 3–6 cm bedding separated by thin (<1–2.5 cm) claystone breaks that appear dark, ~100 m below the Stephen-Eldon contact. (c) Outcrop of shale (calcareous claystone) in the upper Stephen Formation, ~20 m below the Stephen-Eldon contact. In the study area, shales typically form resistant ledges, underlain by recessive thin bedded fine-grained carbonate lithologies. (d) Outcrop of shale in the upper Stephen Formation (~12 m below the Stephen-Eldon contact) showing two prominent dm-scale-deformed slump folds that are pervasive throughout the section and indicate deposition on a sloping surface. (e) Transmitted light micrograph of thin section ofMarrella-bearing interval, showing mm-scale calcareous claystone laminae. Asterisk(*) indicates the position of theMarrella-bearing lamina, ~14.2 m below the Stephen-Eldon contact. (f) Polished slab of fossil-bearing calcareous claystone from within the quarry interval, 2.99–3.08 m below the Stephen-Eldon contact. The prominent 3 cm-thick light-coloured claystone bed at the top of the image bears a particularly diverse and abundant soft-bodied fossil assemblage. Prominent dark-coloured bands at bed tops are enriched in carbonate, as observed in Burgess Shale-type deposits worldwide31. Scale bars, 1 m (a,c); 20 cm (b); 10 cm (d); 1 cm (f) and 2 mm (e). Figure 1: Sedimentary facies. Sedimentary facies of the Stephen Formation at the Marble Canyon locality. ( a , b ) Carbonate mudstone and wackestone facies; ( c – f ) Shale facies. ( a ) Outcrop of carbonate mudstone and wackestone facies showing 2.25 m slump fold in lower field of view, ~30 m above base of the Stephen Formation. ( b ) Outcrop of carbonate mudstone and wackestone facies showing 3–6 cm bedding separated by thin (<1–2.5 cm) claystone breaks that appear dark, ~100 m below the Stephen-Eldon contact. ( c ) Outcrop of shale (calcareous claystone) in the upper Stephen Formation, ~20 m below the Stephen-Eldon contact. In the study area, shales typically form resistant ledges, underlain by recessive thin bedded fine-grained carbonate lithologies. ( d ) Outcrop of shale in the upper Stephen Formation (~12 m below the Stephen-Eldon contact) showing two prominent dm-scale-deformed slump folds that are pervasive throughout the section and indicate deposition on a sloping surface. ( e ) Transmitted light micrograph of thin section of Marrella -bearing interval, showing mm-scale calcareous claystone laminae. Asterisk(*) indicates the position of the Marrella -bearing lamina, ~14.2 m below the Stephen-Eldon contact. ( f ) Polished slab of fossil-bearing calcareous claystone from within the quarry interval, 2.99–3.08 m below the Stephen-Eldon contact. The prominent 3 cm-thick light-coloured claystone bed at the top of the image bears a particularly diverse and abundant soft-bodied fossil assemblage. Prominent dark-coloured bands at bed tops are enriched in carbonate, as observed in Burgess Shale-type deposits worldwide [31] . Scale bars, 1 m ( a , c ); 20 cm ( b ); 10 cm ( d ); 1 cm ( f ) and 2 mm ( e ). 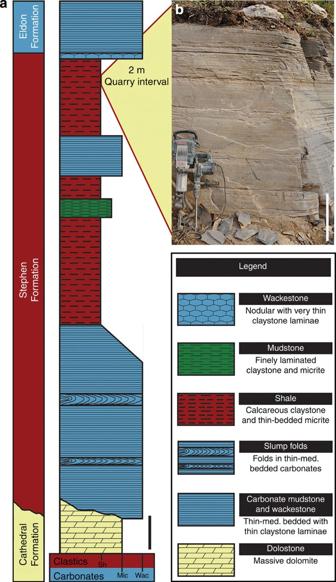Figure 2: The Stephen Formation in the vicinity of Marble Canyon. (a) Idealized stratigraphic section of the Stephen Formation at Marble Canyon, based on detailed measurements at Marble Canyon and observations at Mount Whymper, showing the location of the Marble Canyon fossil assemblage and quarry. (b) Photograph of the main quarry interval, comprising calcareous claystones. Mic, micrite; Sh, shale; Wac, wackestone. Scale bars, 10 m (a); 50 cm (b). Full size image Figure 2: The Stephen Formation in the vicinity of Marble Canyon. ( a ) Idealized stratigraphic section of the Stephen Formation at Marble Canyon, based on detailed measurements at Marble Canyon and observations at Mount Whymper, showing the location of the Marble Canyon fossil assemblage and quarry. ( b ) Photograph of the main quarry interval, comprising calcareous claystones. Mic, micrite; Sh, shale; Wac, wackestone. Scale bars, 10 m ( a ); 50 cm ( b ). Full size image The Marble Canyon assemblage The primary fossil locality ( ca . 2 km east of Marble Canyon) has so far yielded 3,067 specimens ( ca . 80% in situ ) representing a total of 55 taxa ( Supplementary Data 1 ). The fauna encompasses 11 metazoan bodyplans dominated by vagile infaunal, epifaunal and nektobenthic taxa ( Supplementary Fig. 2 ). Two-thirds of the genera present are shared with the Walcott Quarry. These include the arthropods Alalcomenaeus ( Fig. 3a ) , Branchiocaris ( Fig. 3b ), Marrella ( Fig. 3c ) and Naraoia ( Fig. 3d ), the chordate Metaspriggina [14] ( Fig. 3e ), the putative hemichordate Oesia [15] ( Fig. 3f ), the annelid Burgessochaeta ( Fig. 3g ) and the arthropod Molaria ( Fig. 3h ), previously known only rarely from the Walcott Quarry. Liangshanella ( Fig. 3i ) is the most abundant taxon, as in the Walcott Quarry [5] , followed by Oesia ( Fig. 3f ), the mollusc-like Haplophrentis ( Fig. 3k ) and the polychaete Burgessochaeta ( Fig. 3g ). Importantly, two arthropod taxa previously assumed to be endemic to the early Cambrian Chengjiang biota, the problematic Primicaris [16] ( Fig. 3j ) and the nektaspid Misszhouia ( Fig. 3l ), also occur. The presence of these taxa within the Marble Canyon assemblage significantly expands their geographical and temporal ranges, and indicates that their absence from younger Burgess Shale-type assemblages was not the result of endemism or extinction, but was controlled by ecological and taphonomic factors. This finding, together with those from the recently described Early Ordovician Fezouata biota [17] , suggests that the longevity and geographical ranges of soft-bodied Cambrian taxa at both high and low taxonomic ranks may be severely underestimated. 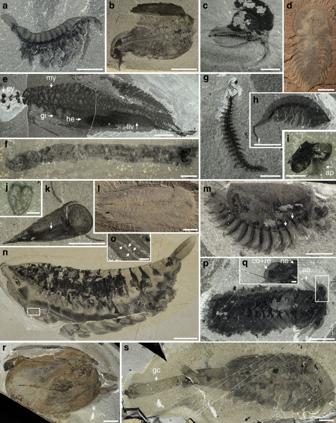Figure 3: Faunal assemblage elements from Marble Canyon. (a) ROM 62967,Alalcomenaeussp. (b) ROM 62968.1,Branchiocarissp. (c) ROM 62969,Marrella splendens. (d) ROM 62970,Naraoiacf.compacta. (e) ROM 62938,Metasprigginacf.walcottiwith preserved eyes and internal organs (composite image of both part and counterpart—stitched images at white lines). (f) ROM 62971,Oesiacf.disjuncta. (g) ROM 62972,Burgessochaetacf.setigera. (h) ROM 62973,Molaria spinifera. (i) ROM 62974.1,Liangshanellacf.burgessensiswith preserved appendages. (j) ROM 62974.2,Primicariscf.larvaformis. (k) ROM 62968.2,Haplophrentiscf.carinatuswith preserved internal organs (arrow). (l) ROM 62975Misszhouiacf.longicaudata. (m) ROM 62976, new isoxyid arthropod (new arthropod B), arrows indicate haemolymph channels. (n,o) ROM 62977, new leanchoiliid (new arthropod L), (n) overall view and (o) close-up showing spinose rami. (p,q) ROM 62978,Mollisonia symmetricawith preserved eyes and appendages, (p) overall view and (q) close-up showing neuropils, cornea and retina. (r) ROM 63014, new bivalved arthropod (new arthropod A). (s) ROM 62974.3,Sidneyia inexpectans, showing possible extruded gut content (arrow). ap, appendages; co+re, cornea+retina; ey, eyes; gc, gut content; gi, gill bars; he, heart; liv, liver; my, myomeres; ne, neuropils. Scale bars, 1 mm (i,j,o,q); 5 mm (a–c,e,g,h,k,m,p) and 10 mm (d,f,l,n,r,s). Figure 3: Faunal assemblage elements from Marble Canyon. ( a ) ROM 62967, Alalcomenaeus sp. ( b ) ROM 62968.1, Branchiocaris sp. ( c ) ROM 62969, Marrella splendens . ( d ) ROM 62970, Naraoia cf. compacta . ( e ) ROM 62938, Metaspriggina cf. walcotti with preserved eyes and internal organs (composite image of both part and counterpart—stitched images at white lines). ( f ) ROM 62971, Oesia cf. disjuncta . ( g ) ROM 62972, Burgessochaeta cf. setigera . ( h ) ROM 62973, Molaria spinifera . ( i ) ROM 62974.1, Liangshanella cf. burgessensis with preserved appendages. ( j ) ROM 62974.2, Primicaris cf. larvaformis . ( k ) ROM 62968.2, Haplophrentis cf. carinatus with preserved internal organs (arrow). ( l ) ROM 62975 Misszhouia cf. longicaudata . ( m ) ROM 62976, new isoxyid arthropod (new arthropod B), arrows indicate haemolymph channels. ( n , o ) ROM 62977, new leanchoiliid (new arthropod L), ( n ) overall view and ( o ) close-up showing spinose rami. ( p , q ) ROM 62978, Mollisonia symmetrica with preserved eyes and appendages, ( p ) overall view and ( q ) close-up showing neuropils, cornea and retina. ( r ) ROM 63014, new bivalved arthropod (new arthropod A). ( s ) ROM 62974.3, Sidneyia inexpectans , showing possible extruded gut content (arrow). ap, appendages; co+re, cornea+retina; ey, eyes; gc, gut content; gi, gill bars; he, heart; liv, liver; my, myomeres; ne, neuropils. Scale bars, 1 mm ( i , j , o , q ); 5 mm ( a – c , e , g , h , k , m , p ) and 10 mm ( d , f , l , n , r , s ). Full size image The arthropod fauna Among the new taxa recovered from the Marble Canyon locality, arthropods are prominent in both diversity and abundance, and include at least 12 new soft-bodied morphotypes. Two of them are ‘great appendage’ stem arthropods, represented by an isoxyid with frontal appendages showing distinct dinocaridid affinities ( Fig. 3m ), and a large leanchoiliid whose typical flagellate ‘short great appendage’ exhibits finely dentate rami in addition to distal claw complex ( Fig. 3n,o ). These new forms will aid in understanding the relationships and disparity of megacheirans [18] , [19] , [20] , [21] and bivalved arthropods [22] , [23] , two groups that continue to play a pivotal role in debates surrounding the early evolution of arthropods. The new evidence emphasizes the predatorial function of leanchoiliid appendages and the likely connections between the dinocaridid and bivalved bodyplans, which have only tentatively been explored so far [24] , but are of critical importance to the evaluation of overall arthropod disparity. Another new bivalved arthropod ( Fig. 3r ) displays sclerotized chelate cephalic appendages, shedding light on the anatomy of the problematic stem arthropod Branchiocaris pretiosa . This confirms that an anterior, post-oral, chelate appendage appeared early, possibly deep within the stem-group of arthropods. The assemblage also yields the first Mollisonia [25] specimen to reveal extensive details of cephalic appendages, together with eyes showing retinal and brain tissues, including putative neuropils ( Fig. 3p,q and inset). Mollisonia was previously known only from elements of the exoskeleton [10] , with soft tissues never before observed. The new material suggests that the neglected taxon Houghtonites [26] actually belongs to Mollisonia , and that this animal was an active benthic predator, based on the presence of large lateral eyes and long cephalic appendages. Fidelity of preservation The consistently high fidelity of preservation in the Marble Canyon material is striking, and expands the range of internal tissues preserved in Cambrian Burgess Shale-type fossils. These include a putative liver and heart in Metaspriggina ( Fig. 3e ), and preservation of branched tridental caeca deep within the limbs of the new isoxyid arthropod ( Fig. 3m ). We also report for the first time the preservation of neural tissues in Burgess Shale material ( Fig. 3p,q ), which, as recently shown for Chengjiang arthropods [27] , promises to yield new phylogenetic information. Additional new anatomical features include a putative gut and indeterminate organs in the enigmatic lophotrochozoan hyolith Haplophrentis ( Fig. 3k ), possible extruded gut content in Sidneyia ( Fig. 3s ), and appendages in Liangshanella ( Fig. 3i ). Appendages in the trilobite Kootenia ( Supplementary Fig. 7 ) are also exceptionally preserved. To date, collection efforts at Marble Canyon have been limited to a single field season of 15 days. Yet, remarkably, the rarefaction curve for Marble Canyon arthropods is markedly steeper than those for arthropods of the Walcott Quarry and Chengjiang assemblages, or for the closely adjacent Stanley Glacier assemblage [10] ( Fig. 4a , Supplementary Table 1 ). Differences in diversity and composition ( Fig. 4b ; Supplementary Table 2 ) between the Marble Canyon assemblage and that of Stanley Glacier are noteworthy, given the close proximity ( ca . 3 km) of the two sites. The density of fossils in the Marble Canyon assemblage, normalized to volume of rock excavated, is significantly higher than that of the Chengjiang or Stanley Glacier localities, and is comparable only to the Walcott Quarry ( Fig. 4c ; Supplementary Data 2 ; Supplementary Note 2 ). Parallel trends in fossil density and diversity indicate that additional collection at Marble Canyon holds great promise for the recovery of new taxa and for enhancing the present understanding of the taxonomic diversity and morphological disparity of the Cambrian fauna. 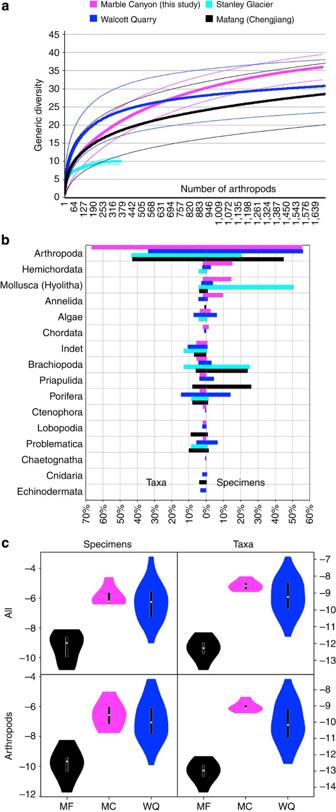Figure 4: Comparison of community attributes and density of specimens between Marble Canyon and other Burgess Shale-type deposits. (a) Rarefied generic diversity curves for arthropods. (b) Relative abundance of taxa and specimens. (c) Violin plots of density. Black bars indicate interquartile range of log density; white dots indicate median of log density; surrounding coloured areas indicate Kernel density plots; MC, Marble Canyon (magenta); MF, Mafang (black), WQ, Walcott Quarry (blue). Figure 4: Comparison of community attributes and density of specimens between Marble Canyon and other Burgess Shale-type deposits. ( a ) Rarefied generic diversity curves for arthropods. ( b ) Relative abundance of taxa and specimens. ( c ) Violin plots of density. Black bars indicate interquartile range of log density; white dots indicate median of log density; surrounding coloured areas indicate Kernel density plots; MC, Marble Canyon (magenta); MF, Mafang (black), WQ, Walcott Quarry (blue). Full size image Patterns in fossil associations point to the recurrence of a similar community-type across the fossil-rich interval ( Supplementary Data 1 ). While this suggests that relatively consistent taphonomic, ecological and environmental conditions prevailed throughout the studied interval, it also highlights important differences in content between Marble Canyon and other Cambrian soft-bodied assemblages elsewhere. Sessile organisms, in particular sponges and brachiopods, which are especially abundant and diverse at the Walcott Quarry [5] and Chengjiang [28] (and to a lesser extent at Stanley Glacier [10] ), are consistently rare at Marble Canyon. Differences in taxonomic composition, as well as in diversity and density, emphasize the role of palaeoenvironment in regulating ecological and taphonomic controls that determined the composition of soft-bodied fossil assemblages, even across small spatial scales. While sampling methodologies, accessibility and collecting efforts vary greatly among Burgess Shale-type deposits, this finding confirms that extraordinarily fossil-rich intervals of the Burgess Shale are neither limited to the type area nor to the lower and middle parts of the formation, which have historically been the focus of investigation. This discovery suggests that the potential of the Burgess Shale to yield exceptional biotas across a spectrum of ecological, environmental and taphonomic gradients remains largely untapped. The particularly large proportion of new taxa that occur within the Marble Canyon assemblage, which lies in close temporal and geographical proximity to the best sampled Cambrian soft-bodied assemblage, the Walcott Quarry, suggests that the present understanding of the diversity and disparity of the earliest complex ecosystems of the Phanerozoic remains in its infancy, and awaits future discoveries. Field collections and repository information All fossil localities visited during the research are protected under the National Parks Act and all fossils and geological samples were collected under a Parks Canada collection and research permit (YNP-2012-12054). The majority of specimens were collected in situ from a 2-m-thick interval (levels −1.75 to −3.5 m below Stephen-Eldon contact −1.5 m 2 in surface area) at the primary quarry site. A minority of specimens come from two fossiliferous intervals below the floor of the quarried interval (−6.5 m, and −14.15 m to −14.25 m, respectively), while about 597 specimens (19% of total) were collected from talus along debris slopes derived primarily from the quarried interval. Of the 2,470 specimens identified from the quarried interval, 85% (2,082) were collected and are now deposited at the Royal Ontario Museum (Invertebrate Palaeontology collections). Shelly fossils from carbonate horizons were collected in the lab via acid maceration (dilute acetic and formic acids). All available exposures of the Stephen Formation in the vicinity of Marble Canyon were measured, sampled and described in cm-scale detail in the field. Observations of sections on Mount Whymper were included in producing a generalized composite section ( Fig. 2 ). Where extensive talus aprons were found to cover portions of the Stephen Formation, a laser rangefinder was used to determine the stratigraphic thickness of the covered interval. Samples were analysed in thin section, polished slab and X-radiograph. Whole-rock chemistry was determined by X-ray fluorescence using a PANalytical Axios X-ray fluorescence at the Pomona College. Bulk and clay mineralogy were determined by X-ray diffraction using a Rigaku Ultima IV diffractometer at the Pomona College. Fossil data sets All fossils were identified to the lowest possible taxonomic rank (usually species) and some specimens were prepared using a micro-engraving tool equipped with a tungsten bit. Owing to lateral variation of individual claystone beds, fossil counts from in situ excavations were pooled into bins spanning 5 cm-thick intervals ( Supplementary Data 1 ). Fossil assemblages used for comparative purposes include the Walcott Quarry (Greater Phyllopod Bed) [5] , [29] , the Mafang locality of the Chengjiang deposit [28] , [30] (fossil assemblages from event beds, only) and the nearby (<3,000 m) Stanley Glacier [10] locality of the ‘thin’ Stephen Formation. Statistical methods EstimateS 9.1.0 ( http://www.viceroy.eeb.uconn.edu/EstimateS/ ) was used to compute individual-based rarefaction curves to allow diversity comparisons between different Burgess Shale assemblages. Density estimates were calculated for intervals with more than 100 specimens (for all phyla) and more than 32 specimens (for arthropods only; Supplementary Data 2 ; Supplementary Note 2 ). Tests and graphics were produced in R ( http://www.r-project.org/ ), and violin plots were drawn using the ‘vioplot’ package. Kruskall–Wallis tests were significant for all comparisons of density among the Mafang, Marble Canyon and Walcott Quarry assemblages. Mann–Whitney (or Wilcoxon) tests between the Mafang assemblage and either the Walcott Quarry assemblage or the Marble Canyon assemblage resulted in P values<10 −4 . For the Walcott Quarry and Marble Canyon localities, P values of Mann–Whitney tests for specimens and taxa in the whole assemblage were 0.43 and 0.14, respectively, thus insignificant and slightly insignificant for a confidence of 95%. When limiting the tests to arthropods, the P value was insignificant for specimen counts (0.36), but slightly significant for taxic counts (0.02). A one-sided version of the test finds that the density of arthropod morphotypes at Marble Canyon is greater than that of the Walcott Quarry ( P value=0.01). Similar tests were run using the data from the Stanley Glacier assemblage; although the number of specimens overall was too low to compare with the others, density estimates were found to be close to that of the Mafang assemblage. How to cite this article: Caron, J.-B. et al. A new phyllopod bed-like assemblage from the Burgess Shale of the Canadian Rockies. Nat. Commun. 5:3210 doi: 10.1038/ncomms4210 (2014).